Probing water micro-solvation in proteins by water catalysed proton-transfer tautomerism Scientists have made tremendous efforts to gain understanding of the water molecules in proteins via indirect measurements such as molecular dynamic simulation and/or probing the polarity of the local environment. Here we present a tryptophan analogue that exhibits remarkable water catalysed proton-transfer properties. The resulting multiple emissions provide unique fingerprints that can be exploited for direct sensing of a site-specific water environment in a protein without disrupting its native structure. Replacing tryptophan with the newly developed tryptophan analogue we sense different water environments surrounding the five tryptophans in human thromboxane A 2 synthase. This development may lead to future research to probe how water molecules affect the folding, structures and activities of proteins. In proteins, water ubiquitously participates in dictating structure and functionality, including protein secondary and tertiary structures, the spontaneous formation of membranes and the recognition of signaling molecules in signal transduction [1] , [2] , [3] . Recent advances have provided more convincing evidence that the water molecules in proteins are key elements in activating bio-functionality such as enzymatic reactions [4] , [5] , [6] , [7] or vice versa , the protein (for example, an antifreeze protein) may affect the organization of water molecules [8] . Probing the water environment of a specifically interesting site in proteins thus may pave a way to understanding the underlying mechanisms and functionality. Unfortunately, although enormous efforts have been made in the characterization of fundamental aqueous hydration phenomena on protein surfaces [9] , [10] , [11] , little insight has been gained into water micro-solvation in protein [12] , [13] . Most of the relevant approaches have focused instead on probing the polarity of the local environment in proteins, particular around the active sites, by means of fluorescence solvatochromism [14] , [15] . To date, Trp in bacterial proteins has been popularly substituted by (7-aza)Trp or in part with (2-aza)Trp , in which the indole moiety in Trp is replaced by 7-azaindole or 2-azaindole ( Fig. 1 ), for either investigating the antimetabolic properties of the Trp isosteres [16] or accessing the local polarity of Trp in proteins with unknown tertiary structures [17] , [18] , [19] , [20] , [21] . Catalysed by protic solvent molecules such as alcohols (for example, methanol), 7-azaindole undergoes solvent-assisted excited-state proton transfer (ESPT), resulting in an N 7 -H tautomer form ( Fig. 2a ) that exhibits green emission (~510 nm) [22] , [23] , [24] . In water, however, the N 7 -H tautomer green emission is virtually non-observable [25] ; this lack has been attributed to the much slower proton-transfer rate constant (~10 9 s −1 ) together with dominant radiation-less deactivation pathways [22] . The photophysical properties of (7-aza)Trp are very similar to those of 7-azaindole , exhibiting essentially no N 7 -H tautomer form emission [16] , [26] , [27] , [28] and thus cannot be used for probing any water-associated photophysical phenomena in proteins. 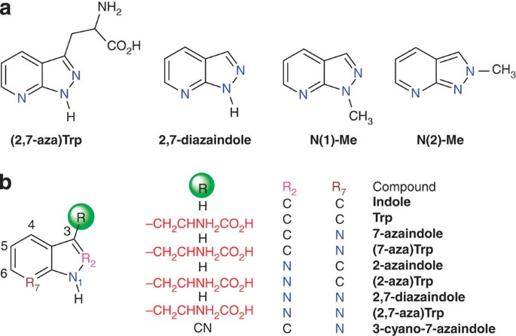Figure 1: The structural formulae of relevant indole and tryptophan derivatives. (a) The chemical structures of(2,7-aza)Trp,2,7-diazaindole,N(1)-MeandN(2)-Me. (b) The chemical structures of various indole and tryptophan analogues. Figure 1: The structural formulae of relevant indole and tryptophan derivatives. ( a ) The chemical structures of (2,7-aza)Trp , 2,7-diazaindole , N(1)-Me and N(2)-Me . ( b ) The chemical structures of various indole and tryptophan analogues. 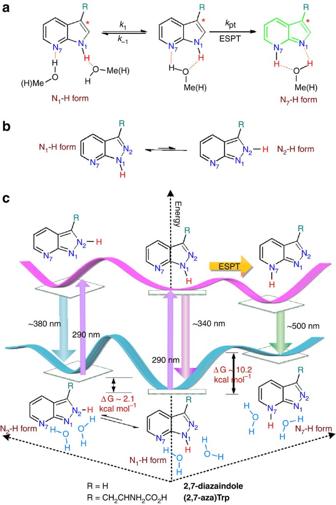Figure 2: Proposed ground and electronically excited states mechanism. (a) The proposed protic solvent catalysed ESPT mechanism for7-azaindoleand its derivatives. The asterisk * indicates the electronically excited state. This mechanism incorporates a fast excited-state equilibrium between polysolvated and 1:1 cyclic hydrogen-bonded N1-H/H2O (or methanol) followed by proton tunnellingkpt22, which has been unambiguously proved by the kinetic deuterium isotope effect29. Under the assumption ofk−1>k1andkpt, the overall ESPT rate constantkrxncan be expressed askrxn=(k1/k−1)kpt. (b) The ground-state equilibrium for2,7-diazaindoleand its derivatives between N1-H form and N2-H form isomers in water. (c) The proposed schematic diagram of a proton-transfer cycle for2,7-diazaindoleand(2,7-aza)Trpin water, in which the barrier and hence potential energy surface are arbitrarily chosen. Full size image Figure 2: Proposed ground and electronically excited states mechanism. ( a ) The proposed protic solvent catalysed ESPT mechanism for 7-azaindole and its derivatives. The asterisk * indicates the electronically excited state. This mechanism incorporates a fast excited-state equilibrium between polysolvated and 1:1 cyclic hydrogen-bonded N 1 -H/H 2 O (or methanol) followed by proton tunnelling k pt [22] , which has been unambiguously proved by the kinetic deuterium isotope effect [29] . Under the assumption of k −1 > k 1 and k pt , the overall ESPT rate constant k rxn can be expressed as k rxn =( k 1 / k −1 ) k pt . ( b ) The ground-state equilibrium for 2,7-diazaindole and its derivatives between N 1 -H form and N 2 -H form isomers in water. ( c ) The proposed schematic diagram of a proton-transfer cycle for 2,7-diazaindole and (2,7-aza)Trp in water, in which the barrier and hence potential energy surface are arbitrarily chosen. Full size image To surpass the limitation of the traditional Trp analogues, we strategically design a new type of aza-Trp by overlapping two azaindole parent moieties, that is, 2-azaindole and 7-azaindole , yielding a new core moiety 2,7-diazaindole ( Fig. 1 ) that is capable of sensing a protein water environment. The underlying concept originates from the molecule 3-cyano-7-azaindole [29] ( Fig. 1 ), in which the cyano electron-withdrawing ability increases hydrogen acidity of the N 1 -H form and hence facilitates the overall ESPT rate in water, rendering an intensive N 7 -H proton-transfer tautomer emission in the green ( Fig. 2a ). For 2,7-diazaindole , the replacement of pyrrole by the pyrazole moiety, in which the N(2) atom acts as an efficient electron-withdrawing group [30] , is expected to increase the N 1 -H proton acidity without perturbing the parent geometry. Using 2,7-diazaindole as the core moiety, we further develop a new Trp analogue, (2,7-aza)Trp ( Fig. 1 ), that exhibits remarkably different properties from classical aza-Trp analogues in that water-assisted proton-transfer isomerization takes place in both the excited and the ground states ( Fig. 2a,b ). The proposed schematic diagram of the proton-transfer cycle for 2,7-diazaindole and (2,7-aza)Trp is depicted in Fig. 2c . Figure 2c unveils the water-catalysed isomerization between the N 1 -H form and the N 2 -H form in the ground state and ESPT for the N 1 -H form in the excited state, as supported by the following firm spectroscopy and dynamics evidence. The associated multiple emissions thus serve as a unique fingerprint for sensing the water environment. The proof of concept is made by the site-specific substitution (2,7-aza)Trp for tryptophan in human thromboxane A 2 synthase (TXAS) to resolve a distinct water environment in various Trp sites of TXAS. Proton-transfer tautomerism Manifested in neutral water (pH=7.0), either (2,7-aza)Trp or 2,7-diazaindole reveals remarkable triply fluorescent bands ( Fig. 3a,b and Table 1 ), consisting of an apparent shoulder at ~330 nm, a peak wavelength at ~370 nm and a much red-shifted emission band maximized at ~500 nm, corresponding to the existence of N 1 -H, N 2 -H and N 7 -H isomers, respectively, in the excited state. The excitation spectra at 335 nm and at the very red edge (for example, 530 nm) of the emission are identical and they also resemble the absorption spectrum ( Supplementary Fig. S1 ). As 2,7-diazaindole and (2,7-aza)Trp were synthesized independently from different methods ( Supplementary Fig. S2 and Supplementary Methods ), the possibility of trace impurities contributing to the triple emission bands can be eliminated. Rather, the triple emission can be well rationalized by the proton-transfer tautomerism in both ground and excited states. Support is provided chemically by the methyl derivatives of 2,7-diazaindole , N(1)-Me and N(2)-Me ( Fig. 1 ), which exhibit prominent emissions at 342 and 367 nm, respectively, in neutral water ( Fig. 3c and Supplementary Fig. S3 ). The emission of N(2)-Me , in view of the peak position (367 nm), is nearly identical to that (370 nm) of 2,7-diazaindole , so the assignment of 2,7-diazaindole 370 nm emission to the N 2 -H isomer appears unambiguous. In addition, given the similarity of its emission peak wavelength (342 nm) to that of N(1)-Me , the 335 nm band in 2,7-diazaindole can reasonably be ascribed to the emission of the N 1 -H isomer. The difference in excitation origins for 335 and 370 nm emission bands ( Supplementary Fig. S1 ) clearly indicates the existence of ground-state equilibrium between N 1 -H and N 2 -H isomers for 2,7-diazaindole ( Fig. 2b ). In accordance with this assignment, we also propose the occurrence of water-catalysed ESPT in the N 1 -H form, forming the N 7 -H isomer, to account for the ~500 nm green emission. Taking account of the structural and spectral similarity, the same assignment of the triple emission should hold true for (2,7-aza)Trp . 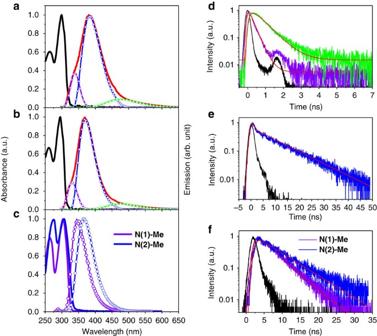Figure 3: Identification of the triple emission bands. (a,b) Absorption (black) and emission spectra (red) of(2,7-aza)Trpare shown inaand2,7-diazaindoleare shown in (b) in neutral water. Further, the decomposed PL spectra are shown (violet, blue and green triangles).λex=290 nm. (c) Absorption and emission spectra ofN(1)-MeandN(2)-Mein neutral water. (d) The emission decay dynamics of(2,7-aza)Trpmonitored at 320 nm (violet) and 540 nm (green). (e) The emission decay dynamics of(2,7-aza)Trpmonitored at 380 nm. (f) The emission decay dynamics ofN(1)-MeandN(2)-Me. The instrument response and the fitting curves are marked in black and red lines, respectively. The residuals of the fit of emission decay dynamics as shown inSupplementary Fig. S8. Figure 3: Identification of the triple emission bands. ( a , b ) Absorption (black) and emission spectra (red) of (2,7-aza)Trp are shown in a and 2,7-diazaindole are shown in ( b ) in neutral water. Further, the decomposed PL spectra are shown (violet, blue and green triangles). λ ex =290 nm. ( c ) Absorption and emission spectra of N(1)-Me and N(2)-Me in neutral water. ( d ) The emission decay dynamics of (2,7-aza)Trp monitored at 320 nm (violet) and 540 nm (green). ( e ) The emission decay dynamics of (2,7-aza)Trp monitored at 380 nm. ( f ) The emission decay dynamics of N(1)-Me and N(2)-Me . The instrument response and the fitting curves are marked in black and red lines, respectively. The residuals of the fit of emission decay dynamics as shown in Supplementary Fig. S8. Full size image Table 1 Photophysical properties. Full size table Firm support for the tautomerism is given by the correlation of relaxation dynamics among emission bands ( Table 1 ). At the short wavelength shoulder of 320 nm, (2,7-aza)Trp exhibits a single decay component of 260 ps in water. At the red edge of the green emission (540 nm), the relaxation dynamics consist of a finite rise component (263 ps) and a decay component with a lifetime of 0.58 ns ( Fig. 3d and Table 1 ). The 263 ps rise dynamic, within experimental uncertainty of ±30 ps, correlates well with the decay of the 340 nm band, supporting the precursor (340 nm band) and successor (500 nm band) type of reaction kinetics and hence the water-assisted ESPT for the N 1 -H isomer. On the other hand, the relaxation dynamics at the peak wavelength of 380 nm consists of an instant, system-response-limited rise time (<60 ps), accompanied by two decay components, one with a small amplitude (~12%), fast decay (265 ps), and a major, long decay component (88%, 10.07 ns, see Fig. 3e ). The former 265 ps component in the 380 nm emission decay, within the experimental error, is identical to 260 ps monitored at 320 nm and thus is assigned to the residue of the N 1 -H emission band. The latter is the population decay of the N 2 -H form emission. The same correlation among the triple emission bands is also resolved for 2,7-diazaindole ( Table 1 ), supporting firmly that both 2,7-diazaindole and (2,7-aza)Trp in water undergo proton-transfer tautomerism in the ground state (N 1 -H/N 2 -H equilibrium) and the excited state (N 1 -H →N 7 -H proton transfer). One fundamental issue lies in the thermodynamics between N 1 -H and N 2 -H isomers in water ( Fig. 2b ). Experimentally, the molar absorption coefficient of N(2)-Me , 5.3 × 10 3 M −1 cm −1 (at 320 nm), was adopted for the N 2 -H isomer of 2,7-diazaindole at 320 nm, a wavelength that is free from N 1 -H form interference. A known concentration of 2,7-diazaindole was prepared, and the N 2 -H/N 1 -H equilibrium constant was measured to be 0.024 (detail in Supplementary Methods ), corresponding to a difference of free energy of 2.2 kcal mol −1 at 298 K. This value is in good agreement with the computational calculations, estimating that the N 2 -H form is 2.1 kcal mol −1 higher in energy than the N 1 -H form for 2,7-diazaindole in water. The same trend is observed but with a rising difference if we consider that less polar solvation by benzene, N 2 -H form, has a higher energy by 6.3 kcal mol −1 for 2,7-diazaindole . We find that this is true with no detectable N 2 -H isomer form emission resolved in organic solvents for 2,7-diazaindole ( Supplementary Figs S4 and S5 ). This proton transfer induced multiple emission in water is remarkable and proves to provide fingerprints for probing a protein water environment. TXAS homology structure and substrate/water gating channel The focus of probing water in proteins is on the cytochrome P450 superfamily because recent advances have generated more convincing data indicating that water molecules have pivotal roles in the organism metabolic pathways in P450s [31] , [32] , [33] . We herein selected the structurally pending TXAS [34] , [35] , [36] , an endoplasmic reticulum membrane protein containing five tryptophans, as a prototype to demonstrate the feasibility of (2,7-aza)Trp in probing water environments. The atypical catalysis without reductase or oxygen and the pathogenesis of major diseases make TXAS of prime interest to elucidate the corresponding structure–function relationship [37] . One recent advance indicates that W65 of TXAS is likely to be in a hydrophobic pocket surrounded by the Phe-cluster, whereas the environment of the other four tryptophans is yet to be determined [38] . A prior molecular dynamic (MD) simulation in this study unveils the spatial arrangement of these five tryptophan residues relative to the haem group and gating channels of TXAS ( Fig. 4a,b ), where W65 residue is on the substrate channel, W133 is located on the aqueduct water channel, W31 lies in the NH 2 -terminal loop and W203 and W446 are close to the protein surface (detail in Supplementary Fig. S6 ). 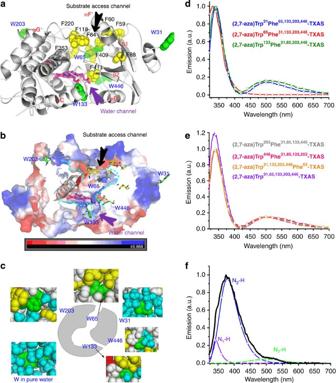Figure 4: MD simulation of TXAS protein and expression of TXAS mutants. (a) TXAS homology structure shows the characteristic P450 fold, illustrating the phenylalanine residues (yellow), five tryptophan positions (green) and haem (stick figures in violet). (b) The solvent-accessible surfaces of the active site cavities calculated using an H probe under an electrostatic potential (ESP) surface with electrophile/nucleophile (blue/red). Proposed gating channels are indicated. (c) The local environment of tryptophan (W) in hydrated TXAS (or water), in which W is shown in green, water is blue, acidic residues are red, hydrophobic residues are yellow and other residues are white. (d,e) Emission spectra of various TXAS mutants excited at 310 nm. The use of two separated figures is to avoid spectral congestion. (f) Emission spectra of denatured(2,7-aza)Trp31,65,133,203,446-TXASand the decomposed PL spectra. Figure 4: MD simulation of TXAS protein and expression of TXAS mutants. ( a ) TXAS homology structure shows the characteristic P450 fold, illustrating the phenylalanine residues (yellow), five tryptophan positions (green) and haem (stick figures in violet). ( b ) The solvent-accessible surfaces of the active site cavities calculated using an H probe under an electrostatic potential (ESP) surface with electrophile/nucleophile (blue/red). Proposed gating channels are indicated. ( c ) The local environment of tryptophan (W) in hydrated TXAS (or water), in which W is shown in green, water is blue, acidic residues are red, hydrophobic residues are yellow and other residues are white. ( d , e ) Emission spectra of various TXAS mutants excited at 310 nm. The use of two separated figures is to avoid spectral congestion. ( f ) Emission spectra of denatured (2,7-aza)Trp 31,65,133,203,446 -TXAS and the decomposed PL spectra. Full size image Expression and analytics of (2,7-aza)Trp -TXAS To examine the relevant tryptophans positions, TXAS mutants were synthesized in Trp-auxotrophic Escherichia coli cells [39] , and they proved to be capable of co-translational incorporation by site-specifically replacing Trp residues with (2,7-aza)Trp (see Supplementary Methods ). Fig. 4d and e depict the fluorescence spectra of various mutants. As for single (2,7-aza)Trp substitution at W31, W133, W203 and W446, the resulting (2,7-aza)Trp 31 Phe 65,133,203,446 -TXAS , (2,7-aza)Trp 133 Phe 31,65,203,446 -TXAS , (2,7-aza)Trp 203 Phe 31,65,133,446 -TXAS and (2,7-aza)Trp 446 Phe 31,65,133,203 -TXAS exhibit prominent, well-resolved dual emissions maximized at ~340 nm (N 1 -H) and ~505 nm (N 7 -H), indicating the occurrence of N 1 -H to N 7 -H proton-transfer in the excited state. By taking advantage of the MD simulations, we were able to examine the proximal environment around various Trp sites of TXAS. We found no relevant amino acids forming direct H-bonds with the mutant ( (2,7-aza)Trp s, also eliminated the possibility of the ESPT catalysed from the protic residues. Therefore, the results ensure the water-catalysed ESPT for the single (2,7-aza)Trp substitution at each of four Trp sites in TXAS. For (2,7-aza)Trp substitution at W31, W203 and W446, time-resolved measurement monitored at 350 nm clearly reveals a major 0.28–0.30 ns (±0.03) decay component, which correlates well with the rise time of the ~505 nm emission band of 0.30–0.32 ns (±0.03) ( Table 1 ). Both spectroscopy and dynamics data are reminiscent of the water-catalysed ESPT of the (2,7-aza)Trp N 1 -H isomer in water. As shown in Fig. 4d , the observed dual emission also guarantees the occurrence of water-catalysed ESPT for single (2,7-aza)Trp -substituted TXAS mutants at W133. However, compared with that of W31, the slight increase of green tautomer emission intensity and the associated faster rate of ESPT (0.21±0.03 ns, Table 1 ) may imply its difference in a water environment. Supported by water titration experiments for 7-azaindole [25] , [40] , the breakdown of bulk water clusters may facilitate the rate of ESPT. Accordingly, we tentatively propose that there is a reduced water density region at the W133 site ( cf . W31). The results of MD simulation elaborated in a later section seem to support this viewpoint. In sharp contrast, for the single (2,7-aza)Trp substitution at W65, the resulting (2,7-aza)Trp 65 Phe 31,133,203,446 -TXAS exhibits solely an emission band maximized at 332 nm with a long lifetime of ~1.55 ns ( Fig. 4d and Table 1 ). The apparent lack of a 500 nm emission band speaks to the nature of the prohibition of ESPT at the W65 position in TXAS, concluding the deficiency of water molecules surrounding the proximity of the W65 site. Support is further given by the full (2,7-aza)Trp substitution of all five tryptophan residues in the expression of (2,7-aza)Trp 31,65,133,203,446 -TXAS mutant, which exhibits well-resolved dual emissions maximized at ~340 and 507 nm as well ( Fig. 4e ). Notice that the intensity ratio for the 340 nm emission band versus the 500 nm emission band is slightly higher than that of quadruple (2,7-aza)Trp substitution of (2,7-aza)Trp 31,133,203,446 Phe 65 -TXAS mutant, indicating the increase of 340 nm emission due to the prohibition of ESPT in (2,7-aza)Trp65. Statistically, however, the mixture of incomplete substitution of (2,7-aza)Trp at any Trp sites is likely to occur in (2,7-aza)Trp 31,65,133,203,446 -TXAS . Therefore, the corresponding quantitative spectral analysis is not possible. Nevertheless, the selected excitation wavelength at 310 nm should be virtually free of absorption by trace Trp residues. Unambiguously, the results present a unique feature, that the position at W65 is subject to a water-deficient microenvironment wherein the lack of surrounding water molecules prohibits ESPT, resulting in a solely normal N 1 -H form 340 nm emission. The other four tryptophans (W31, W133, W203 and W446) in TXAS are in a water-accessible microenvironment that catalyses ESPT, resulting in an N 7 -H tautomer green emission. Importantly, unlike the triple emission of dissolved (2,7-aza)Trp in water, all native (2,7-aza)Trp -TXAS mutants reveal an absence of N 2 -H form 380 nm emission ( cf . Figs 3a and 4d,e ). This seems to describe the vital folding structure of a solvated protein. In a native folding, the associated framework in protein (TXAS) is different from the unfolding residues exposed in the bulk water solution, in which the N 2 -H isomer is solvated and stabilized at the sufficient water hydration level. Moreover, the TXAS conformer polarity may not be high enough to stabilize the N 2 -H isomer, being similar to the lack of population of N 2 -H isomer in organic solvents ( vide supra , see Supplementary Fig. S4 , in methanol). Firm support of this viewpoint is given by the reappearance of the N 2 -H form 380 nm emission upon denaturing of (2,7-aza)Trp 31,65,133,203,446 -TXAS variants ( Fig. 4f ). The lack of N 2 -H isomer emission thus indicates that none of the (2,7-aza)Trp in (2,7-aza)Trp -TXAS mutants are bulk water-solvated, and so the Trps in wild-type TXAS, due to the structural similarity. Explicit solvent MD simulations on both wild-type TXAS and (2,7-aza)Trp -replaced TXAS have been performed and showed no detectable differences in terms of the solvated homology structure. The results indicate that the TXAS matrices are dynamically coupled to the hydration water by a relay-type of hydrogen-bonding configuration ( Fig. 4c ). This, together with the close-up inspections of the hydrogen-bonding configurations for each (2,7-aza)Trp -replaced tryptophans in TXAS ( Supplementary Fig. S6 ), draws two important remarks. First, there are clearly no water molecules surrounding the W65 site. Second, except for W65, water micro-solvation does exist for all other (2,7-aza)Trp . When compared with explicit water MD simulations, a locally fluctuating density profile is revealed (detail in Supplementary Methods and Supplementary Fig. S7 ), so it seems to be apparent that fewer trapped water molecules associate with the W133 site. Both results are consistent with the experimental observation ( vide supra ). The combination of experimental and MD approaches thus proves the feasibility of (2,7-aza)Trp in probing the micro-solvation structures in protein. As manifested by explicit solvent MD simulations, two distinct channels are identified as the substrate access channel (W65 locus) and the aqueduct water channel (W133 locus) in protein TXAS ( Fig. 4b ). The associated faster rate of ESPT in (2,7-aza)Trp133 seems to specify the destination of hydration water behaviours between the protein surface and aqueduct water channel in protein. Also worthy of note is the hydrophobic region located on the substrate channel; this region, with phenylalanine residues (Phe60, Phe64, Phe127, Phe220, Phe409 and Phe411) and W65, forms a ‘Phe-cluster’. This distinctive Phe-cluster and hydrophobic residues on the TXAS substrate channel [38] result in a less polar and water-deficient microenvironment at the active site, which is in stark contrast to its counter-enzyme prostacyclin synthase (PGIS), which has greater water accessibility to the active haem site [39] , [41] . This prediction is firmly supported by the prohibition of ESPT in (2,7-aza)Trp65. The location of the Phe-cluster results in a gating conformation of the active site of TXAS. MD simulations also reveal that conformational movement of the Phe-cluster residues could open/close the channel and consequently increase/decrease the volume of the active site of TXAS. We hypothesize that this relevant locus of the ‘Phe-cluster’ is crucial in gating different ligand/water access in an early step of allowance to the active haem site. In summary, we have developed a new tryptophan analogue, (2,7-aza)Trp , which undergoes water-catalysed proton-transfer tautomerism in both ground and excited states, giving a multiple emission that is sensitive to the water environment. Incorporating (2,7-aza)Trp into human TXAS, we then demonstrate for the first time the feasibility to probe water molecules surrounding in proteins. Manifested by explicit solvent MD simulation, (2,7-aza)Trp -TXAS mutant maintains its parent wild-type TXAS structure. Exploiting co-translational (2,7-aza)Trp as a probe, correlation between these biocompatible probing spectra and a water micro-solvation environment has been established, thereby identifying specific tryptophan locations on TXAS. The incorporation of (2,7-aza)Trp into TXAS proves (2,7-aza)Trp to be a novel optical probe that allows transmission of its surrounding water environment into unique fluorescence spectral features. In combination with in-depth MD simulation, future quantitative correlation for the ESPT dynamics versus number/orientation of water molecules is feasible, showing different hydration environments between the substrate access channel, aqueduct water channel and protein surface in, for example, TXAS. The superb water-sensing capability in terms of ESPT and ground-state N 1 -H/N 2 -H equilibrium thus provides an unprecedented tool for probing the water environment in bio-systems on a structural basis. General synthesis and characterization Full experimental details, synthesis and characterization for all compounds, computational methodology, growth and induction of bacteria are included in the Supplementary Methods . Steady-state and time-resolved fluorescence spectroscopy Steady-state absorption and emission spectra were recorded on a Hitachi (U-3310) spectrophotometer and an Edinburgh (FS920) fluorimeter, respectively. Both wavelength-dependent excitation and emission response of the fluorimeter had been calibrated. Time-resolved spectroscopic measurements were carried out by means previously reported elsewhere in detail [42] , [43] . Briefly, nanosecond (ns) lifetime studies were performed with a time-correlated single-photon counting (TCSPC, Edinburgh FL 900), using a hydrogen-filled lamp as the excitation source. The emission decays were analysed by the sum of exponential functions as below, which allows partial elimination of instrument time broadening and thus renders a temporal resolution of ~300 ps. To achieve a faster time resolution, studies were also performed using a TCSPC system (Edinburgh OB-900L) coupled with an excitation light from the third harmonic generation (THG, at 306 nm) of pulse-selected femtosecond laser pulses at 920 nm (90 fs, Tsunami and Model 3980 pulse picker, Spectra-Physics). The temporal resolution is ~60 ps. Data were analysed by using the nonlinear least-squares procedure in combination with an iterative convolution method. Tautomer structure calculations The theoretical approach used the Second-Order Approximate Coupled-Cluster method (CC2) [44] together with a resolution-of-the-identity technique to enhance performance. All atoms were employed using correlation-consistent basis sets of double-ζ quality with the diffuse and polarization functions (aug-cc-pVDZ) [45] . All calculations incorporated the solvation (COSMO model) [46] for ground-state geometry optimization. All the theoretical calculations were performed with the TURBOMOLE programme package (version 6.3) [47] , [48] , [49] , [50] . Thermodynamics of various isomers in different solvents were calculated using the DFT approach (B3LYP 6–311+g(d,p)) incorporating a continuum solvation model (Gaussian 09) [51] . How to cite this article: Shen, J.-Y. et al . Probing water micro-solvation in proteins by water catalysed proton-transfer tautomerism. Nat. Commun. 4:2611 doi: 10.1038/ncomms3611 (2013).